In vivoimaging and histochemistry are combined in the cryosection labelling and intravital microscopy technique Intravital microscopy has been used extensively to study dynamic processes in the context of a living animal; however, only a limited number of fluorescent probes and mouse models are available. By contrast, many dyes and antibodies exist for the immuno-labelling of fixed tissue. Here we report a method that combines the advantages of histochemistry and in vivo imaging by correlating cryosection labelling with corresponding intravital microscopy images (CLIM). Using CLIM, we find that the presence of CD3 + T cells correlates with mammary tumour cell migration. When CD4 + and CD8 + T-cell subsets are depleted, reduced tumour cell migration is observed. From these data we conclude that CLIM is a powerful tool to correlate intravital microscopy data with cryosection labelling data. Immunohistochemistry of fixed tissue sections has been used extensively to study the composition of tissues using an almost unlimited number of commercially available antibodies. Nevertheless, immunohistochemistry can only provide a snapshot of often dynamic tissue. By contrast, high-resolution intravital microscopy (IVM), a technique by which individual cells inside a living animal can be visualized, enables the visualization of cellular processes in real time [1] , [2] , [3] , [4] . However, IVM depends on a limited number of available fluorescent probes and mouse models [5] , [6] . The limitations of both techniques hamper the study of the full complexity of tissues. Ideally, one would combine the advantages of both IVM and immunohistochemistry: first image cells in vivo and then retrace areas of interest in histological sections. Correlative microscopy, such as correlative light-electron microscopy, has been used to combine the advantages of two microscopy techniques [7] . We have recently reported a simple and effective correlative microscopy approach to mark and track single cells in living tissue based on photo-conversion of the fluorescent protein Dendra2 (ref. 8 ). Although we are able to identify red-marked cells in immunohistochemical sections, the drawback of this technique is that cells need to express photo-convertible proteins. As the vast majority of fluorescent mouse models for intravital imaging lack Dendra2 expression, it is desirable to develop a correlative microscopy technique without the requirement of photo-convertible proteins. Landmarks, such as blood vessels or collagen fibres, have been used to retrace IVM imaging areas over multiple days [3] , [9] , [10] , but they are by far too abundant to correlate IVM images with immunohistochemical sections. In vitro , near-infrared branding has successfully been used to create fiducial marks in fixed tissue, which can be used as a guide to correlate previously imaged structures in electron microscopy images [11] . Here we report the development of a correlative microscopy method termed cryosection labelling and intravital microscopy (CLIM), which is based on infrared light, to create fiducial marks in the tissue of living animals that can be used to correlate dynamic intravital images with the images of sections that are fluorescently labelled by immunohistochemistry. Using CLIM we find that CD4 + and CD8 + T cells support the migration of tumour cells in mouse-invasive lobular carcinomas (mILCs). A two-photon laser can generate photo-tattoos in vivo Using a femtosecond pulsed titanium−sapphire laser tuned at 800 nm, we created a three-dimensional highly intense autofluorescent fiducial mark in a defined region of the tumorigenic tissue of a living mouse, which we refer to as photo-tattoo ( Fig. 1a ). Although photo-tattooing executed at low power (<300 mW at the sample) created photo-tattoos without visible damage on tissue such as the type I collagen fibres, high-power fiducial marks (>600 mW at the sample) did create visible tissue damage ( Fig. 1b ; the large red arrows point to damaged collagen fibres). As neutrophils are the first cells to infiltrate damaged tissue, we imaged their recruitment directly after photo-tattooing. Indeed, photo-tattooing at high laser power resulted in damaged vasculature and subsequent neutrophil recruitment ( Fig. 1c and Supplementary Fig. S1a ). We observed that 13 min after photo-tattooing the first neutrophils were being recruited to the tattoo ( Fig. 1c,d and Supplementary Fig. S1b ). This indicates that, when a tissue is isolated and fixed within 13 min after photo-tattooing, the photo-tattoo has not recruited immune cells yet. Therefore, tissues were isolated within 10 min after the photo-tattoo was placed and then instantly snap-frozen or formalin fixed and subsequently snap-frozen. For experiments that study local immune activation that precedes the infiltration of immune cells (for example, release of cytokines), photo-tattooing after whole animal fixation by transcardial perfusion is preferable. Indeed, we were able to photo-tattoo formalin-fixed tissues ( Fig. 1e ). 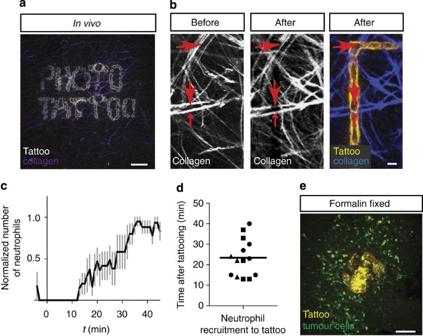Figure 1: Photo-tattooing creates fiducial marksin vivo. (a) Photo-tattoo of a mammary tumour created by a multiphoton laser tuned at 800 nm. Scale bar, 100 μm. (b) Damaged (large arrow) and non-damaged (small arrow) type I collagen fibres (white in left image and blue in right image) before and after photo-tattooing. Scale bar, 20 μm. (c,d) TAMRA-SE-labelled neutrophils were adoptively transferred into recipient mice. The recruitment of neutrophils upon photo-tattooing the liver (with low power) was visualized by IVM. (c) The number of neutrophils present in the tattooed area plotted against time. The neutrophil numbers were normalized to the highest number for every experiment. The tattoo was made att=0. Tattoos (n=5) in three different mice. Error bars, s.e.m. (d) The time between the generation of the tattoo and the entrance of neutrophils in the tattoo was measured and plotted in the graph.n=13 neutrophils in five tattoos in three different mice. Symbols represent different mice. (e) A representative image of a photo-tattoo that was made in a formalin-fixed tumour (n=3). Scale bar, 100 μm. Figure 1: Photo-tattooing creates fiducial marks in vivo . ( a ) Photo-tattoo of a mammary tumour created by a multiphoton laser tuned at 800 nm. Scale bar, 100 μm. ( b ) Damaged (large arrow) and non-damaged (small arrow) type I collagen fibres (white in left image and blue in right image) before and after photo-tattooing. Scale bar, 20 μm. ( c , d ) TAMRA-SE-labelled neutrophils were adoptively transferred into recipient mice. The recruitment of neutrophils upon photo-tattooing the liver (with low power) was visualized by IVM. ( c ) The number of neutrophils present in the tattooed area plotted against time. The neutrophil numbers were normalized to the highest number for every experiment. The tattoo was made at t =0. Tattoos ( n =5) in three different mice. Error bars, s.e.m. ( d ) The time between the generation of the tattoo and the entrance of neutrophils in the tattoo was measured and plotted in the graph. n =13 neutrophils in five tattoos in three different mice. Symbols represent different mice. ( e ) A representative image of a photo-tattoo that was made in a formalin-fixed tumour ( n =3). Scale bar, 100 μm. Full size image Photo-tattooing of serum components As intravital imaging is performed in a wide range of organs, we tested whether photo-tattooing can generate fiducial marks in various tissues ( Fig. 2a ). Interestingly, we observed variations in the efficiency of photo-tattooing among different tissues. For example, in tumours with a heterogeneous vascularization, we observed varying success rates between 50 and 100%. High efficiencies were found in highly vascularized organs, such as in the liver and spleen. Moreover, we found that photo-tattooing is highly efficient in tissue containing leaking vasculature ( Fig. 2b ). Furthermore, in contrast to flowing vessels ( Fig. 2c ), where tattooed molecules will be carried away from the tattooed site, the tattoo is efficient in vessels where the blood flow has stalled (stalled vessels are occasionally present in tumour tissue ( Fig. 2d )). These data suggest that a component of the blood may be required for creating fiducial marks by photo-tattooing. To further specify which fraction of the blood is responsible for the photo-tattoo marks, we separated the blood and found that only the serum and not the white blood cell (WBC) fraction could be photo-tattooed ( Fig. 2e ). Interestingly, photo-tattooed serum contained multiple fluorescent components, because differential emission spectra were detected when different excitation wavelengths were used to record the emission spectrum ( Fig. 2f ). Therefore, we conclude that photo-tattooing enhances the autofluorescence of multiple serum components. 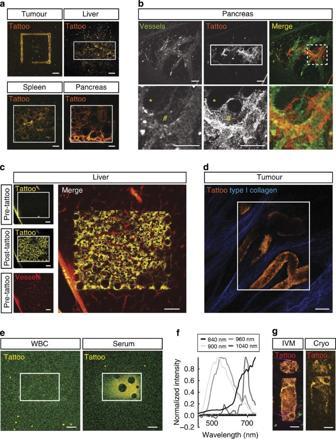Figure 2: A multiple serum component photo-tattoo. (a) Tattoos were generated with high power in the liver, spleen, pancreas and mammary tumour tissues using a multiphoton laser tuned at 800 nm. Yellow represents the tattoo.n≥3 mice. Scale bars, 100 μm. (b) Upper images: a tattoo was generated (the squared region with the solid line) within the pancreas. The dashed square indicates the region shown with high magnification in the lower panels. Green illustrates the vasculature, red the tattoo. Lower images: the region where high-molecular-weight Rhodamin-Dextran (2,000 kDa) leaked out of the vasculature is indicated with ‘#’ and the non-leaky area with ‘*’. Note that the leaky area is more efficiently tattooed than the non-leaky area. Scale bars, 100 μm. (c) A region of the pancreas was imaged before and after photo-tattooing with high laser power. The vasculature (fluorescent dextran) is shown in red, and in yellow the tattoo. Scale bar, 100 μm. (d) A photo-tattoo was generated using low laser power in a region of a tumour with a few stalled vessels as indicated by the white square. The tattoo is seen in yellow, and type I collagen in blue. Note that only in the tattooed region the vessels are highlighted by the tattoo. Scale bar, 100 μm. (e) Photo-tattooing of the WBC fraction and the serum fraction (serum) isolated from mice (representative images from ≥9 tattoos). White box indicates the tattooed area. Scale bars, 100 μm. (f) Emission spectra of the photo-tattoo after excitation with various wavelengths. (g) A tattoo (red) made after IVM was retraced in a 16-μm-thick cryosection (Cryo). Scale bar, 20 μm. Figure 2: A multiple serum component photo-tattoo. ( a ) Tattoos were generated with high power in the liver, spleen, pancreas and mammary tumour tissues using a multiphoton laser tuned at 800 nm. Yellow represents the tattoo. n ≥3 mice. Scale bars, 100 μm. ( b ) Upper images: a tattoo was generated (the squared region with the solid line) within the pancreas. The dashed square indicates the region shown with high magnification in the lower panels. Green illustrates the vasculature, red the tattoo. Lower images: the region where high-molecular-weight Rhodamin-Dextran (2,000 kDa) leaked out of the vasculature is indicated with ‘#’ and the non-leaky area with ‘*’. Note that the leaky area is more efficiently tattooed than the non-leaky area. Scale bars, 100 μm. ( c ) A region of the pancreas was imaged before and after photo-tattooing with high laser power. The vasculature (fluorescent dextran) is shown in red, and in yellow the tattoo. Scale bar, 100 μm. ( d ) A photo-tattoo was generated using low laser power in a region of a tumour with a few stalled vessels as indicated by the white square. The tattoo is seen in yellow, and type I collagen in blue. Note that only in the tattooed region the vessels are highlighted by the tattoo. Scale bar, 100 μm. ( e ) Photo-tattooing of the WBC fraction and the serum fraction (serum) isolated from mice (representative images from ≥9 tattoos). White box indicates the tattooed area. Scale bars, 100 μm. ( f ) Emission spectra of the photo-tattoo after excitation with various wavelengths. ( g ) A tattoo (red) made after IVM was retraced in a 16-μm-thick cryosection (Cryo). Scale bar, 20 μm. Full size image Photo-tattoo used to retrace IVM areas in cryosections To employ photo-tattoos as fiducial landmarks to correlate cryosection labelling with intravital microscopy (CLIM) ( Fig. 2g ), we marked the IVM-imaged areas of mammary tumours ( Fig. 3a and Supplementary Movie 1 ) with photo-tattoos ( Fig. 3b ). The tattoos were placed one field of view away from the area of interest. After harvesting, the tissues were frozen in such a way that the intravitally imaged region was pressed flat against a tissue mould ( Fig. 4 ). Next, using a cryotome, consecutive cryosections of the first millimeter of the imaged region were cut ( Fig. 3c ) and collected on a microscopy slide. Although the tattoos are still visible in rehydrated slides, we searched for tattoos in non-rehydrated slides ( Fig. 3d ), because rehydration decreased the intensity of the tattoos. If cryosections are cut in exactly the same angle as the thin optical IVM sections, the tattoo can be found within one 16-μm-thick cryosection. However, in the vast majority of experiments the angle did not match exactly ( Fig. 3c ), and the optical IVM section was distributed over several cryosections ( Fig. 3e ). Thus, the IVM optical section needed to be reconstructed from several cryosections ( Fig. 3f ). After matching the cryosections to the IVM images ( Fig. 3g ), we rehydrated the cryoslides and we determined the degree of freezing-mediated tissue shrinkage ( Fig. 3h ). On average, the tattoo was 8.1%±1.1 smaller in cryosections compared with IVM images ( Fig. 3 dot plot). Next, we determined in the IVM images the coordinates of the cells of interest relative to the tattoo ( Fig. 3i ), and used the shrinkage-corrected coordinates ( Fig. 3j ) to retrace the same cells in the cryosections ( Fig. 3k ). As an additional control for retracing, we checked whether the shape of the retraced cells matched in the IVM image and the cryosection image ( Fig. 3l ). Using this method, we were able to retrace intravitally imaged regions in immuno-stained cryosections ( Fig. 3 , Supplementary Fig. S2 ). These data show that the photo-tattooed regions used for CLIM are effective fiducial marks to correlate intravital images and cryosections. 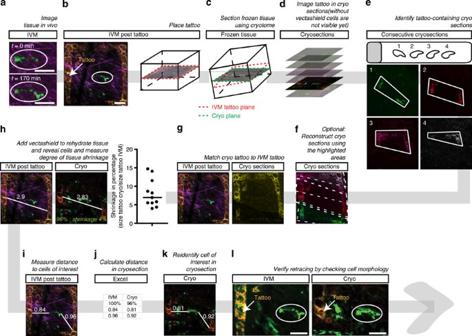Figure 3: CLIM pipeline to re-identify intravitally imaged regions in cryosections. (a) Cells of interest (encircled) are imaged intravitally. (b) After the IVM session, a photo-tattoo is placed. (c) Imaged tissue is isolated, frozen and sectioned by a cryotome. Note that when the angle of the cryosections is not equal to the angle of the optical IVM section, the tattoo will be distributed over multiple consecutive cryosections. (d) Consecutive cryosections in the first 1 mm of tissue are transferred to glass slides and imaged. (e–g) The tattoo is reconstructed when distributed over multiple cryosections and matched with the IVM image. (h) The degree of tissue shrinkage is determined in rehydrated tissues (for typical values, see the right graph). (i) The coordinates of the cells of interest relative to the tattoo are determined in the IVM image. (j,k) Shrinkage-corrected coordinates are used to retrace the cells of interest in the cryosection. (l) The successful retracing is confirmed by comparing cell shapes. Scale bar, 80 μm. Figure 3: CLIM pipeline to re-identify intravitally imaged regions in cryosections. ( a ) Cells of interest (encircled) are imaged intravitally. ( b ) After the IVM session, a photo-tattoo is placed. ( c ) Imaged tissue is isolated, frozen and sectioned by a cryotome. Note that when the angle of the cryosections is not equal to the angle of the optical IVM section, the tattoo will be distributed over multiple consecutive cryosections. ( d ) Consecutive cryosections in the first 1 mm of tissue are transferred to glass slides and imaged. ( e – g ) The tattoo is reconstructed when distributed over multiple cryosections and matched with the IVM image. ( h ) The degree of tissue shrinkage is determined in rehydrated tissues (for typical values, see the right graph). ( i ) The coordinates of the cells of interest relative to the tattoo are determined in the IVM image. ( j , k ) Shrinkage-corrected coordinates are used to retrace the cells of interest in the cryosection. ( l ) The successful retracing is confirmed by comparing cell shapes. Scale bar, 80 μm. 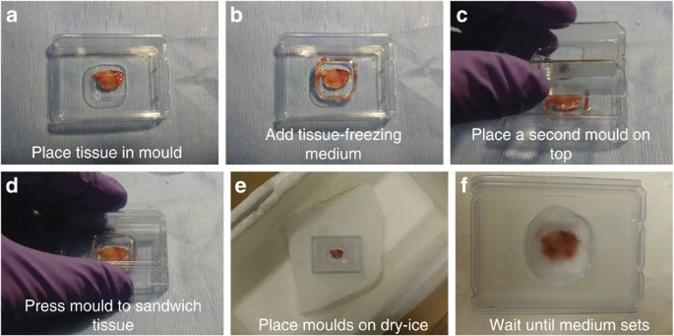Figure 4: Freezing procedure of intravitally imaged tissue. (a–f) After the IVM session, the isolated tissue was placed in a tissue mould with the imaged region facing down (a). Next, tissue-freezing medium was added (b) and a second tissue mould was placed on top of the tissue (c). The tissue was flattened by pressing the two moulds (d). Next, the moulds were placed on dry-ice (e) to solidify the freezing medium (f). Full size image Figure 4: Freezing procedure of intravitally imaged tissue. ( a – f ) After the IVM session, the isolated tissue was placed in a tissue mould with the imaged region facing down ( a ). Next, tissue-freezing medium was added ( b ) and a second tissue mould was placed on top of the tissue ( c ). The tissue was flattened by pressing the two moulds ( d ). Next, the moulds were placed on dry-ice ( e ) to solidify the freezing medium ( f ). Full size image T cells support migration of tumour cells It has been shown that the migration and metastasis of tumour cells is dependent on and influenced by the tumour microenvironment. Here, we utilized CLIM to identify factors in the microenvironment that drive the migration of tumour cells in mILCs. Orthotopic injection of mILC-1 cells into female 129P2/OlaHsd;FVB/n mice leads to mILCs [12] . We intravitally imaged these mammary tumours for ~3 h and found that the migratory behaviour of tumour cells was very heterogeneous; in some regions of the tumour >10% of the cells were migratory, whereas in other regions of the same tumour none of the tumour cells migrated. For example, the top panel of Fig. 5a and Supplementary Movie 2 show a region where the number of migratory cells is small, whereas the lower panel shows a region of the same tumour where the number of migratory cells is large. To measure migration in imaged regions, we quantified the number of non-colocalizing pixels between the first and last images of the time series and correlated that to the total tumour cell area, which confirms high migration in the bottom panel and low migration in the top panel ( Fig. 5a ). Next, we tried to identify the microenvironmental component that correlates with the differential cell behaviour in these two regions. One of these potential factors, CD4 + T cells, has been shown to have a role in metastasis in the PyMT and Neu breast cancer model, but not in a NeuT breast cancer model [13] , [14] , [15] . To correlate the presence of CD4 + and CD8 + T cells with the metastatic behaviour of mILC breast cancer cells, we used our newly developed CLIM method to determine the role of T cells specifically during tumour cell migration, one of the first steps of metastasis. After retracing the intravitally imaged cells in cryosections using CLIM, we stained the sections for the pan T-cell marker CD3. Interestingly, we found that in regions with high tumour cell migration a high number of CD3 + T cells were present, whereas in regions with very little tumour cell migration only a few CD3 + T cells were present ( Fig. 5a ). These data suggest that the presence of T cells is correlated with tumour cell migration. To confirm this correlation and to further characterize the responsible T-cell subset, we injected mice for two weeks with T-cell-depleting antibodies for either CD4 + or CD8 + T cells, and confirmed that this indeed led to a loss of the respective T cells in the mILC tumours ( Fig. 5b ). Next, we performed intravital imaging on tumours in which either CD4 + or CD8 + T cells were depleted. As suggested by our CLIM data, we indeed found that migration was greatly diminished when mice were treated for 2 weeks with CD4- or CD8-depleting antibodies ( Fig. 5c ). Therefore, we conclude that the migration of mILC-1 tumour cells is linked to the presence of CD4 + and CD8 + T cells. 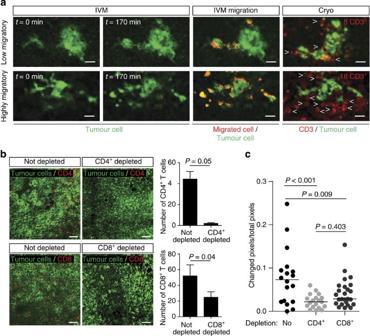Figure 5: CLIM identifies T cells as important contributors to mILC tumour cell migration. (a) A mILC tumour region with a low amount of migratory signals (top panel) and a region with a high amount of migratory signals (bottom panel) were retraced in cryosections and stained for CD3+T cells. Pixels that have been changed between the images oft=0 and 170 min are indicated with orange. In the cryo-image, the CD3 signal is red and the arrowheads point to some of the T cells. Note the high number of T cells in the migrating area, and the low number of T cells in the non-migratory area. Scale bar, 15 μm. (Representative images ofn=3 experiments, each performed in three mice.) (b) Left: images showing positive CD4+or CD8+T cells in 16-μm stained tumour sections of non-depleted, CD4+-depleted or CD8+-depleted mice. Right: average number of T cells in tumour sections in the conditions as indicated.P-values were obtained using an unpaired Mann–WhitneyU-test.n≥5 areas in at least three different mice. Error bars, s.e.m. Scale bar, 100 μm. (c) In IVM movies of mILC, tumour cell migration (the ratio of changed cell area—indicated as orange ina—to the total cell area) was measured in non-depleted control mice, CD4 Ab-depleted and CD8 Ab-depleted mice (n>17 positions from at least three mice per condition). A one-way ANOVA with Bonferroni’s multiple comparison correction was used to determine if there was a significant difference between the different conditions. Median is indicated. Figure 5: CLIM identifies T cells as important contributors to mILC tumour cell migration. ( a ) A mILC tumour region with a low amount of migratory signals (top panel) and a region with a high amount of migratory signals (bottom panel) were retraced in cryosections and stained for CD3 + T cells. Pixels that have been changed between the images of t =0 and 170 min are indicated with orange. In the cryo-image, the CD3 signal is red and the arrowheads point to some of the T cells. Note the high number of T cells in the migrating area, and the low number of T cells in the non-migratory area. Scale bar, 15 μm. (Representative images of n =3 experiments, each performed in three mice.) ( b ) Left: images showing positive CD4 + or CD8 + T cells in 16-μm stained tumour sections of non-depleted, CD4 + -depleted or CD8 + -depleted mice. Right: average number of T cells in tumour sections in the conditions as indicated. P -values were obtained using an unpaired Mann–Whitney U- test. n ≥5 areas in at least three different mice. Error bars, s.e.m. Scale bar, 100 μm. ( c ) In IVM movies of mILC, tumour cell migration (the ratio of changed cell area—indicated as orange in a —to the total cell area) was measured in non-depleted control mice, CD4 Ab-depleted and CD8 Ab-depleted mice ( n >17 positions from at least three mice per condition). A one-way ANOVA with Bonferroni’s multiple comparison correction was used to determine if there was a significant difference between the different conditions. Median is indicated. Full size image Taken together, we have developed a correlative microscopy method, CLIM, to correlate intravitally imaged regions in immunohistochemical cryosections. For CLIM endogenous fluorescence is used, and therefore it does not require time-consuming and expensive mouse genetics and it can be applied to a wide variety of tissues that are intravitally imaged. Using CLIM it will be possible to use a wide variety of antibodies to screen for factors whose presence is correlated to a specific behaviour in vivo . This may help to identify new components that influence in vivo cell behaviour such as migration. Furthermore, if combined with laser capture microdissection and transcardial fixation, it may be possible to dissect tissue of which the in vivo history is known and which can be used for further analyses such as mass spectrometry [16] , microarray analysis [17] or genomic sequencing [18] . Primary invasive lobular carcinoma tumours are a heterogeneous population of cells that includes cancer cells and a variety of immune cells such as T cells and macrophages [19] . Here, we have shown that the presence of T cells is linked to mILC tumour cell migration. T cells may facilitate tumour cell migration directly, for example via secretion of RANKL, which is known to enhance the metastatic potential of RANK-expressing tumour cells [15] , or indirectly, for example by recruiting migration-inducing M2 macrophages, as was shown for the PyMT model [14] . Future research should determine the exact mechanisms by which T cells enhance mILC tumour cell migration. Taken together, these findings emphasize the power of CLIM to correlate IVM data with cryosection labelling data. DNA constructs and transfections Dendra2 was cloned from the pDendra2 (Evrogen) into a pLV.CMV construct (a kind gift from P. Derksen, University Medical Center Utrecht). mILC-1 cells were transduced using a standard lentiviral transduction protocol. Afterwards, cells were three times sorted on fluorescence by flow cytometry to create a stable cell line. Cell lines mILC-1 tumour cells were derived from mILC tumours of K14cre;Cdh1 F/F ;Trp53 F/F mice as described in Derksen et al. [12] They were cultured in Dulbecco’s Modified Eagle’s Medium (DMEM) F12+GlutaMAX (GIBCO, Invitrogen Life Technologies) supplemented with 5% (v/v) fetal bovine serum (Sigma), 5 ng ml −1 insulin, 5 ng ml −1 epidermal growth factor, 100 μg ml −1 streptomycin and 100 U ml −1 penicillin (all Invitrogen Life Technologies). 4T1 cells (obtained from Eric Daanen) were cultured in DMEM (GIBCO, Invitrogen Life Technology) supplemented with 5% (v/v) fetal bovine serum (Sigma), 100 μg ml −1 streptomycin and 100 U ml −1 penicillin (all Invitrogen Life Technologies). Cells were kept at 37 °C in a humidified atmosphere containing 5% CO 2 . Antibodies and reagents CD4 and CD8 antibodies (both 1 mg ml −1 ) were kindly provided by Karin de Visser. Rabbit anti-mouse CD3 antibody was obtained from Thermo Scientific (Clone SP7, dilution 1:200); rat anti-mouse CD4 eFluor660 (GK1.5, dilution 1:100) and rat anti-mouse CD8 eFluor660 (53–6.7, dilution 1:100) antibodies were obtained from eBioscience. Mouse models All experiments were carried out in accordance with the guidelines of the Animal Welfare Committee of the Royal Netherlands Academy of Arts and Sciences, The Netherlands. Mice were housed under standard laboratory conditions and received food and water ad libitum . 29P2/OlaHsd and FVB/n (The Jackson Laboratory) mice were crossed to obtain female 129P2/OlaHsd;FVB/n mice. If necessary, mice were injected in the fourth mammary fat pad with 5 × 10 5 mILC-1 Dendra2 or 4T1 tumour cells at 8 weeks of age. Intravital imaging was performed at 6–10 weeks after injection, when the tumour was on average 64 mm 2 . Adoptive transfer of neutrophils and subsequent intravital imaging were performed in BALB/c mice between 7 weeks and 6 months of age. Intravital imaging Mice were sedated using isoflurane inhalation anaesthesia (1.5–2% v/v isoflurane in O 2 ), and shaved before surgery. The mouse was placed on an inlay containing a hole covered with a coverslip. A skinflap procedure was performed as described [20] to expose the tumour. In short, the skin surrounding the tumour was excised while leaving the lateral side and large blood vessels intact. The animal was placed with its belly downwards on an inlay containing a hole with a coverslip on top. The tumour was exposed by fixing the skinflap to the inlay (using tape), with the tumour facing the coverslip. When imaging abdominal organs, a midline incision through skin and abdominal wall was made. The organ of interest was extracorporated using phosphate-buffered saline (PBS)-drenched cotton swabs and placed on top of the cover slip. The mouse was taped to the inset to ensure a stable position of the mouse and organ. A wet cotton gauze (drenched in PBS) was placed next to the incision and covered with parafilm to prevent dehydration. Next, the inlay was placed within a custom-designed imaging box. The isoflurane was introduced through a facemask, and ventilated by an outlet. The imaging box and microscope were kept at 32 °C by a climate chamber. Imaging was performed on an inverted Leica TCS SP5 AOBS two-photon microscope with a chameleon Ti:Sapphire pumped optical parametric oscillator (Coherent Inc.). Photo-tattooing Photo-tattoos were placed at the end of an intravital imaging experiment. First, an XYZ position next to an area of interest was chosen. The chameleon Ti:Sapphire two-photon laser was tuned to 800 nm and the laser power was adjusted to 200–600 mW. In a defined region of interest a continuous scan was started (usually with a zoom of > × 2). The development of the tattoo was followed over time using two non-descanned detectors (NDDs): NDD3 (500–550 nm) and NDD4 (560–650 nm). Continuous scanning was performed for various times between 5 s and 5 min depending on the tissue being tattooed. After scanning the tattoo could be excited using two-photon microscopy as explained in ‘Equipment and settings’, and could be detected by the eye through the eye-piece. Acquisition of emission spectra of photo-tattoos The fluorescent emission spectra of photo-tattoos were acquired on a Leica SP5 multiphoton microscope. Excitation wavelength was set as 840, 960, 900 or 1,040 nm. Emission spectra were collected on an internal descanned detector. A stack of images was acquired, where the detection bandwidth of 10 nm was shifted a few micrometres to the red wavelength for every subsequent image. From these series, the emission spectra were measured using imageJ software. Re-identification of photo-tattoos in cryosections After photo-tattooing, the area of the organ that was imaged (was visible through the coverslip) was resected and placed with the imaged-side down in a tissue mould. Tissue-freezing medium (Leica Microsystems Nussloch GmbH) was added until the entire organ was covered and a second tissue mould was placed on top. To ensure that the photo-tattooed area was flat, the tissue was sandwiched in between the two tissue moulds. The entire preparation was placed on top of a flat piece of dry-ice until the tissue-freezing medium had solidified. The tissue was sectioned using a Leica cryotome CM 3050 by placing the tissue on a holder and by ensuring the angle of sectioning was parallel to the tissue-freezing medium surface. Tissue sections of size 16 μm were cut, and every section was collected by placing them on tissue slides. Dry tissue sections were then scanned for tattoos using a widefield microscope. After identification of the tattoos, the slides were stored at −20 °C, or used for CLIM. If immunostaining was performed after CLIM, sections were placed in PBS for 1 h to dissolve the VECTASHIELD hard+set mounting medium. Then the slides were rehydrated, acetone fixed and immunostained. Immunostaining was done according to a standard immunohistochemistry protocol. Neutrophil recruitment Neutrophils were purified from mouse bone marrow by isotonic Percoll gradient centrifugation. Briefly, BALB/c mice were euthanized and the femurs and tibia from both hind legs were removed. The bone marrow was flushed with wash buffer (1 × HBSS+0.5% heat-inactivated FBS+2 mM EDTA). Red blood cells were lysed using NH 4 Cl lysis buffer (155 mM NH 4 Cl+10 mM KHCO 3 +0.1 mM EDTA in H 2 O). Neutrophils were separated from the remaining cells by layering on a three-step (50, 55 and 80%) isotonic Percoll gradient (GE Healthcare). Neutrophils at the 55–80% interface were removed, washed and labelled with carboxytetramethylrhodamine-succinimidyl ester (TAMRA-SE) (Invitrogen). Labelled neutrophils were injected intravenously into mice bearing an abdominal imaging window on their liver as described previously [21] . Neutrophil recruitment was monitored 5 min pre-tattooing and in 45 min time-lapse movies post-tattooing with a time resolution of 1 min. The values were normalized to the highest number of neutrophils found for every time series. Isolation of WBC/serum The WBC and serum fractions were isolated using histopaque according to the manufacturer’s protocol. The various fractions were placed on a microscopy slide and covered by a cover slip. Antibody depletion Mice received three intraperitoneal injections with the depleting antibody. First injection (day 0), 400 μg; second injection (day 3), 100 μg; and third injection (day 5), 100 μg. Imaging was performed on day 7. The depletion was verified by staining of tumour sections with CD4- or CD8-eFluor660 antibodies. Equipment and settings All images were recorded on a Leica TCS SP5 AOBS two-photon microscope with a chameleon Ti:Sapphire pumped optical parametric oscillator (Coherent Inc.). The microscope is equipped with four NDDs: NDD1 (<455 nm), NDD2 (455–490 nm), NDD3 (500–550 nm) and NDD4 (560–650 nm). Different wavelengths between 700 and 1,150 nm were used for excitation. Second harmonic generation signal was obtained with a wavelength of 960 nm and detected with NDD2. Dendra2 was excited with a wavelength of 960 nm and Dextran 2,000 kD Rhodamine with a wavelength of 840 nm. Intravitally, the photo-tattoo was excited with a wavelength of 840, 900, 960 or 1,040 nm, and detected with NDD4, NDD3 and NDD4, NDD3 and NDD4, and NDD4, respectively. In cryosections, the photo-tattoo was excited with a 405, 488, 495 or 633 laser, and detected between 450 and 490, 498 and 580, 505 and 580, and 643 and 700 nm, respectively. All images were acquired with a × 25 (HCX IRAPO N.A.0.95 WD 2.5 mm) water objective or a × 20 (HCX IRAPO N.A.0.70 WD 0.5 mm) dry objective using a zoom of × 1.7 or × 1, and a bit depth of 12 bits. All pictures were processed using ImageJ software (NIH, Bethesda, MD, www.nih.gov ); pictures were contrasted (if necessary and only in a linear manner), smoothed (if necessary), cropped (if necessary), rotated (if necessary) and converted from 12-bit to 8-bit RGB (Red Green Blue) colour images. How to cite this article: Ritsma, L. et al. In vivo imaging and histochemistry are combined in the cryosection labelling and intravital microscopy technique. Nat. Commun. 4:2366 doi: 10.1038/ncomms3366 (2013).